Ultrafast isomerization initiated by X-ray core ionization Rapid proton migration is a key process in hydrocarbon photochemistry. Charge migration and subsequent proton motion can mitigate radiation damage when heavier atoms absorb X-rays. If rapid enough, this can improve the fidelity of diffract-before-destroy measurements of biomolecular structure at X-ray-free electron lasers. Here we study X-ray-initiated isomerization of acetylene, a model for proton dynamics in hydrocarbons. Our time-resolved measurements capture the transient motion of protons following X-ray ionization of carbon K-shell electrons. We Coulomb-explode the molecule with a second precisely delayed X-ray pulse and then record all the fragment momenta. These snapshots at different delays are combined into a ‘molecular movie’ of the evolving molecule, which shows substantial proton redistribution within the first 12 fs. We conclude that significant proton motion occurs on a timescale comparable to the Auger relaxation that refills the K-shell vacancy. Proton migration in the acetylene dication has received significant attention as a model for understanding isomerization driven by nonadiabatic electron–nuclear interactions in more complex organic materials. Measurements reported by Osipov et al. [1] , [2] indicate that, when initiated by X-ray core ionization, this isomerization can occur on a timescale shorter than 60 fs. This ultrafast rate was unexpected based on the predicted barrier heights in the electronic states populated in relaxation on core ionization [3] , [4] . We investigated this process in a time-resolved X-ray pump/X-ray probe experiment at Linac Coherent Light Source (LCLS), a free electron laser (FEL) X-ray source at SLAC National Accelerator Laboratory. This new technique allows direct probing of the isomerization in the time domain. X-ray FELs can produce intense femtosecond pulses of coherent X-rays. These light sources have been employed for molecular and material science, as well as structural biology [5] , [6] , [7] , [8] , [9] , [10] , [11] , [12] , [13] , [14] , [15] . Current and future X-ray FELs plan to deliver ultrashort X-ray pulses with sufficiently high intensity to collect diffraction images of selected targets in a single shot. This prospect of nearly instantaneous diffraction-before-destruction is motivating a dedicated research effort at X-ray FELs [16] , [17] , [18] . Single-particle diffraction requires an X-ray pulse duration shorter than the timescale associated with the radiation damage [5] , [6] , [19] , [20] , [21] . Core ionization and subsequent Auger decay in intense X-ray fields creates a highly charged molecule that eventually falls apart by Coulomb repulsion. The small mass of protons makes intramolecular proton migration the fastest nuclear response to the significant disruption of the electronic structure caused by the X-ray ionization. The acetylene dication is the smallest hydrocarbon that can isomerize and is thus a prototype for investigations of the electronic–nuclear nonadiabatic interactions that underlie basic unimolecular isomerization and radiation damage of biological material, relevant for diffraction-before-destruction techniques and in vivo radio-oncology [22] . The nonadiabatic interactions that hinder the separation of the electronic and nuclear motion in molecules under certain conditions cause the Born-Oppenheimer approximation to break down and require advanced quantum computational techniques for treatment [23] . Isomerization of acetylene (HCCH) to form vinylidene (H 2 CC) has been studied in the neutral molecule, as well as singly and doubly charged acetylene ions [1] , [2] , [24] , [25] , [26] , [27] , [28] , [29] , [30] , [31] , [32] , [33] , [34] , [35] , [36] . Acetylene cations are important not only as a model for molecular dynamics and radiation damage investigations, but also in a range of applications, from plasma devices [37] , combustion [38] , semiconductor manufacturing [39] and to understanding planetary atmospheres [40] . Isomerization of the dication has been investigated in synchrotron experiments [1] , [2] , [27] , [28] , [34] . Osipov et al. [1] , [2] performed ion–ion–photoelectron and ion–ion–Auger electron coincidence measurements to study the fragmentation of the dication formed on core ionization of acetylene. These measurements place an upper limit of 60 fs on the time for the X-ray-initiated isomerization [1] , [2] . Osipov et al. proposed that the isomerization occurs on the lowest singlet state of the dication (see Fig. 1 ), although participation of the 1 Δ g state could not be ruled out [2] . Calculations [3] , [4] predict the barrier for the isomerization on the potential energy surface to be 2.3 eV. At the same time, the vibrational excitation of the acetylene dication after Auger decay is expected to be smaller than the barrier height [2] . This would imply isomerization times on the picosecond timescale according to the transition-state theory [4] . The mechanism of the unexpectedly fast isomerization could not be probed by the measurements reported in refs 1 , 2 , because they were not time resolved. This process has been studied in time-resolved optical laser experiments coupled with three- and four-particle coincident detection [30] , [32] , [33] , [36] . 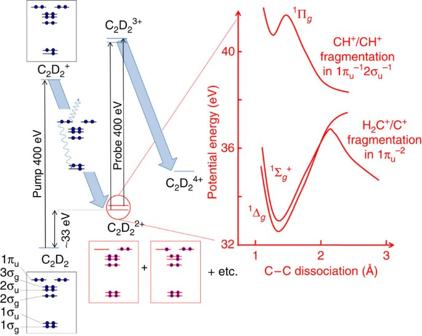Figure 1: Excitation scheme. Acetylene dication states discussed in the text are given after ref.2. The first X-ray pulse core ionizes the acetylene molecule, which relaxes by Auger electron emission. This process populates dicationic states, some of which are shown on the right hand side. According to ref.2isomerization to vinylidene occurs on thepotential energy surface, while acetylene-like fragmentation occurs in an excited configuration. On a variable delay the second X-ray pulse further core-ionizes the dication. Quadruply charged ion, formed on the loss of the second Auger electron, dissociates and the fragment momenta are analysed as described in the text. Figure 1: Excitation scheme. Acetylene dication states discussed in the text are given after ref. 2 . The first X-ray pulse core ionizes the acetylene molecule, which relaxes by Auger electron emission. This process populates dicationic states, some of which are shown on the right hand side. According to ref. 2 isomerization to vinylidene occurs on the potential energy surface, while acetylene-like fragmentation occurs in an excited configuration. On a variable delay the second X-ray pulse further core-ionizes the dication. Quadruply charged ion, formed on the loss of the second Auger electron, dissociates and the fragment momenta are analysed as described in the text. Full size image Optical laser experiments find that deuterium migrates to form vinylidene on a timescale of ∼ 90 fs when strong-field 800 nm radiation initiates isomerization. In the singly charged ion the ultrafast isomerization is not launched with 800 nm radiation, but has been demonstrated to proceed from the excited A state [26] , [35] . Core ionization, which was employed in the current work for initiating isomerization, occurs in the weak-field regime, unlike the strong-field 800 nm experiments. Core ionization, followed by Auger relaxation, results in a different distribution of dicationic states and a different degree of vibrational excitation than strong-field ionization. The isomerization mechanism can differ between these two cases. To measure the ultrafast timescale of this prototypical X-ray-initiated isomerization, we perform a time-resolved X-ray pump/X-ray probe experiment at LCLS that directly detects the geometry change in . rather than is employed to eliminate potential background sources of protons from water or other contaminants. Although the two molecules have the same electronic structure, if the isomerization rate is limited by the nuclear masses, one would expect both the particle velocity and the rate of the tunnelling through the barrier to be slower in compared with . Our measurements indicate that the isomerization in the deuterated acetylene dication already begins in the first 12 fs following core ionization. This finding is consistent with a non-static geometry before the Auger transition. As suggested by Gadea et al. [41] , when lighter nuclei are involved, molecular geometry can begin to evolve during the core-hole lifetime. This geometry change during the core-hole excitation, which is typically neglected in the analysis of core-ionization experiments, implies that transition-state theory applied to the potential energy surface of the dication alone is insufficient to account for the ultrafast proton migration [4] . This result will inform realistic models of radiation damage of biomaterials in single-molecule diffraction experiments at FEL X-ray sources [5] , [6] , [42] , [43] . Strategy for the ultrafast X-ray probe In the experiment the first X-ray pulse (400 eV, up to 10 fs long, 100 μJ per pulse) ionizes the carbon K-shell in the molecule, which, in the dominant relaxation channel, subsequently loses a second electron via Auger decay (see Fig. 1 ). The dication is created in a non-stationary state, a superposition of many electronic states, each with a different degree of vibrational excitation. The relaxation that follows initiates the geometrical change that can lead to isomerization and molecular breakup. On a variable delay a second X-ray pulse, with the same characteristics as the first one, probes the instantaneous geometry in the relaxing dication by further core ionization and Auger decay. The result is , which has no bound states [44] . The final charge state of 4+ is nearly impossible to reach via absorption of only one X-ray photon, and is indicative of the time-dependent pump-probe dynamics. Its dissociation fragments reveal the geometry of the molecule at the probe delay time. Molecules that absorb two photons from one X-ray pulse and fragment as a tetracation contribute to a time-independent background. Alternative direct and shake ionization paths that involve the L-shell of carbon typically lead to a different final charge state than the 4+ channel. A combination of a loss of three electrons through a shake process in one step, and a loss of one electron in L-shell ionization in another step, would lead to the final state of 4+. This combination is at least two orders of magnitude less likely than the excitation path discussed in the text. Measurement of the momenta of all molecular fragments, in coincidence, as a function of time delay between the two X-ray pulses gives information about the evolution of the instantaneous molecular geometry during the relaxation of the dication. On the basis of total charge and momentum conservation we can separate the ion coincidences arising from the fragmentation of the tetracation from those arising from the background or the fragmentation of the molecule in other charge states. More details of the experiment and data processing can be found in Methods section. Differentiation between acetylene and vinylidene To fully characterize the instantaneous molecular geometry, we must detect each of the four ion fragments produced on dissociation. In this report, we discuss the time evolution of the fragmentation channel in which two deuterons and two singly charged carbon ions originating from a single molecule were detected. The conditions applied to identify the true C + /C + /D + /D + coincidences are discussed in Methods section. To classify the four-particle coincidences as arising from the vinylidene or the acetylene isomer, we define the angle θ : which is the angle that a deuteron momentum makes with the effective C–C axis. Here the effective C–C axis is defined by the momenta of the two heavier fragments, as the direction of the vector in a moving frame tied to the centre of mass of the two heavier particles. Vectors and refer to the carbon and deuteron momenta, respectively. To ensure that the vector is well-defined in a given fragmentation event, we also require that the two C + ions depart with momenta pointing close to 180° from each other. In other words: where has the value of 1.0 rad (see Supplementary Fig. 1 in for the distribution of ). The angle θ enables us to classify the C + /C + /D + /D + coincidences as ‘vinylidene-like’ (‘V-like’ further in the text) if (both deuteron momenta reside on the same side of the plane that divides the carbon–carbon axis). The remaining coincidences, when , (two deuteron momenta on opposite sides of this plane) are referred to as ‘acetylene-like’ or ‘A-like’. The angle θ is an approximate measure of the CCD angle, because the momenta in the four-particle fragmentation are not required to point along the instantaneous directions of the molecular bonds. We point out that our labels ‘A’ and ‘V’ are defined by the directions of the particle momenta, regardless of the order in which the bonds break. Relative rotation of CCD + fragments can also lead to an apparent V-like angle θ . As both the experiment reported here and that reported in ref. 2 used non-resonant core ionization, the same dicationic state distribution is created in both experiments. By measuring the energy of the Auger electrons simultaneously, Osipov et al. [2] concluded that the CH + /CH + channel originates from excited electronic configurations of the dication, while the channel comes from the configuration (see Fig. 1 ). In addition, they find that fragments are detected exclusively in coincidence with highest-energy Auger electrons, which indicates that isomerization does not occur in dicationic states that arise from excited configurations. We populate the same dicationic states as Osipov et al. That means that, although many excited dicationic states contribute to the C + /C + /D + /D + dissociation channel in our experiment, the signal indicative of isomerization arises from the same states as discussed in the ref. 2 . Plots of the angle θ track the differences between the V and A channels. In Fig. 2 we plot the total kinetic energy release (KER) summed over all four fragments as a function of θ integrated over the time delay. The right half of the plot contains the A-like coincidences and the left half the V-like ones. It is apparent in Fig. 2 that mean KER and the KER distribution width display a dependence on the angle θ . The mean KER value for the V-like population is several electronvolts lower than that of the A-like population. Osipov et al. report a higher KER for the CH + /CH + channel compared with that of the CH 2 + /C + channel in the fragmentation of the . The same experiment reported a broader distribution of the KER in the CH + /CH + channel compared with that of the channel [2] . Although the energetic ordering does not have to be preserved in four-body fragmentation, Fig. 2 indicates that in the case of acetylene this order is not altered. The broad distribution of the KER in the A-like channel implies that the dication is formed with significant vibrational excitation following Auger relaxation. 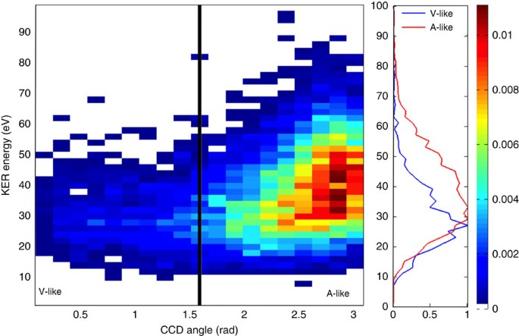Figure 2: Acetylene/vinylidene differentiation. The distribution of all C+/C+/D+/D+coincidences is plotted as a function of the total kinetic energy release and the angleθ. The plot contains the data integrated over all time delays. The solid black line divides the vinylidene-like geometries (left) and acetylene-like ones (right). The data for the two isomers display a difference in both the peak KER and the width of its distribution, as shown on the right hand side. Figure 2: Acetylene/vinylidene differentiation. The distribution of all C + /C + /D + /D + coincidences is plotted as a function of the total kinetic energy release and the angle θ . The plot contains the data integrated over all time delays. The solid black line divides the vinylidene-like geometries (left) and acetylene-like ones (right). The data for the two isomers display a difference in both the peak KER and the width of its distribution, as shown on the right hand side. 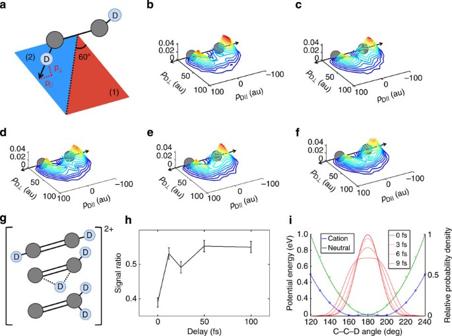Figure 3: Temporal evolution of the deuteron momenta. The directions parallel and perpendicular to the C–C axis are defined ina. The measurements were done at 0 fs (b), 12 fs (c), 25 fs (d), 50 fs (e) and 100 fs (f). While the deuteron momentum distribution indicates localization in CD bond length and CCD angle at 0 fs, at longer time delays both the average CCD bending angle and the width of geometry distributions increase. Acetylene and vinylidene isomers, as well as the transition state are shown schematically ing. The broadening of the distribution leads to an increase in the signal in region 1 (shaded red ina) and a disappearance in region 2 (shaded blue ina). Region (1) shaded red inapertains to the combinations of the deuteron momentum components where 0°<tan−1(p||/p⊥)<60° , while the region (2) pertains to 60°<tan−1(p||/p⊥)<120°. The ratio of the signal in the region 1 to that in the region 2 is shown inh. The relative error inhis given by the inverse of the square root of the number of coincidences at each time delay. Potential energy surfaces for theground state of neutral acetylene (green) and thestate of core-ionized cation (blue; thestate of the core-ionized cation is almost isoenergetic) along the bending mode are shown ini, together with the broadening of the wavefunction on the timescale of the Auger relaxation. More details about the calculation is given inSupplementary Fig. 2. Full size image Time dependence in the measurement Figure 3 shows a dependence of the deuteron momentum distribution on the time delay between the two pulses. The deuteron momenta are represented in the centre of mass frame of the two carbon ions. We choose the x axis along the C–C momentum difference and the component of the deuteron momentum along this direction is referred to as the parallel component. We use to define the y axis. Its component parallel to the C–C relative momentum is selected to be the y axis. The component of the deuteron momentum along the y axis is referred to as the perpendicular component. We always select the direction of the x axis so that the deuteron with the smaller y component has a negative x component. With these axes the migrating deuteron is on the left and we can monitor the temporal evolution in the distribution of the average CCD molecular angle, which is reflected in the evolution of the deuteron moment distribution as shown in Fig. 3 . Figure 3: Temporal evolution of the deuteron momenta. The directions parallel and perpendicular to the C–C axis are defined in a . The measurements were done at 0 fs ( b ), 12 fs ( c ), 25 fs ( d ), 50 fs ( e ) and 100 fs ( f ). While the deuteron momentum distribution indicates localization in CD bond length and CCD angle at 0 fs, at longer time delays both the average CCD bending angle and the width of geometry distributions increase. Acetylene and vinylidene isomers, as well as the transition state are shown schematically in g . The broadening of the distribution leads to an increase in the signal in region 1 (shaded red in a ) and a disappearance in region 2 (shaded blue in a ). Region (1) shaded red in a pertains to the combinations of the deuteron momentum components where 0°< tan −1 ( p || / p ⊥ )<60° , while the region (2) pertains to 60°<tan −1 ( p || / p ⊥ )<120°. The ratio of the signal in the region 1 to that in the region 2 is shown in h . The relative error in h is given by the inverse of the square root of the number of coincidences at each time delay. Potential energy surfaces for the ground state of neutral acetylene (green) and the state of core-ionized cation (blue; the state of the core-ionized cation is almost isoenergetic) along the bending mode are shown in i , together with the broadening of the wavefunction on the timescale of the Auger relaxation. More details about the calculation is given in Supplementary Fig. 2 . Full size image The momentum distribution in Fig. 3 indicates that the maximum localization in both the magnitude and the angle of the deuteron momentum occurs at zero time delay ( Fig. 3b ). This localization is particularly pronounced for the deuteron with the smaller perpendicular component of the momentum. This observation suggests greater localization in the CD bond length and CCD angle at zero time delay. Such localization is consistent with an initial single deprotonation step in near-linear geometry. The averaged CCD angle indicates that the Auger relaxation produces vibrationally hot acetylene, predominantly sampled at turning points of the CCD bending mode. An unequal momentum peak height of the two deuterons and, hence, an unequal distribution width is already apparent at the nominal zero time delay, as expected for vibrationally hot sample. As the migrating deuteron on the left is more delocalized, its momentum peak height is smaller. At larger delays, an increase in both the average CCD angle, as well as the spread of the CCD angles, is evident. Although this spreading in the CCD angle is most significant at longest time delay of 100 fs where almost complete loss of localization of the deuteron momentum angle and magnitude is observed ( Fig. 3f ), it is important to note that the angle increase is already observable at the earliest non-zero time delay (12 fs) in the experiment ( Fig. 3c ). To characterize the broadening of the proton momentum distribution, in Fig. 3h , we plot the time dependence of the ratio of the signal in the region (1) to that in the area in the vicinity of the left carbon (region (2), as illustrated in Fig. 3a ). Time dependence of this ratio indicates that the bending motion towards the isomerization barrier is already launched on the shortest timescale sampled by our experiment. This is consistent with the upper limit for the isomerization time reported in ref. 1 . The increase in the bending angle at 12 fs, compared with 0 fs, is followed by a discernible decrease at 25 fs. This could be a signature of a vibrational coherence, since 12 fs corresponds to one-quarter of the period of the antisymmetric bending mode in the state of the acetylene dication [3] . Similar evolution of the bending angle is observed in the analysis of the events where only three fragments, C + , C + and D + , are detected (see Supplementary Fig. 2 ). We note that the cross correlation between the two X-ray pulses can affect the zero-delay point. When both pulses arrive at the same time, it is possible for a core-ionized molecule to absorb the second X-ray photon before the Auger relaxation occurs. This results in double-core-hole formation, which for acetylene could be localized on the same carbon or distributed between the two carbon atoms. This manuscript concentrates on the channels in which equal sharing of the charge occurs among the four fragments, which may suppress detection of signatures of double-core-hole relaxation. To understand the fast onset of the isomerization, which is already apparent at the shortest delay in our experiment, we discuss in more detail the dynamics in the core-ionized acetylene ion before Auger relaxation. When one of the carbon atoms becomes core ionized, the sudden change in the Coulomb field at the site of the deuterium atom bound to that carbon atom initiates motion of that deuteron. In other words, if the core-excited singly charged ion is created in a non-stationary state, it will begin to relax via a geometry change. This relaxation begins before interruption by the Auger relaxation. The extent of the geometry change during the core excitation depends on the core-hole lifetime and is typically neglected in considering core ionization [2] , [4] , [41] . This approximation is better for cases of core excitation of nuclei with fast Auger relaxation rates, as well as for heavier nuclei that experience unscreened fields. With light species, such as deuterons or protons, this geometry change during the ∼ 6 fs carbon 1 s core-hole lifetime [45] may not be negligible. Gadea et al. [41] suggested that a similar mechanism may play a role in core-to-valence excitation of acetylene. Thus, if the motion on the potential energy surface of the core-excited lasts sufficiently long, the deuterium atom adjacent to the core-excited carbon can acquire a non-negligible momentum that persists after the Auger relaxation occurs. In addition, the dication is created in an initial geometry different from that of the neutral ground state acetylene. Both the alteration in the geometry and the initial momentum can modify the path towards isomerization. Therefore, even if isomerization is incomplete during the core-hole lifetime, the molecule can be launched on the path towards isomerization before the Auger transition occurs. Similarly, the wavepacket evolves on a mostly coulombic potential in the trication before the second Auger relaxation. To test the possibility that molecular geometry changes during the core-hole lifetime, we calculated the potential energy as a function of the bending angle in the highly excited singly charged acetylene ion (see Fig. 3i and Supplementary Fig. 3 ). The potential energy plot shows that the vibrational constant for the bending mode decreases in the core-excited singly charged ion, compared with the neutral. The anharmonicity of the potential energy for the core-ionized cation leads to broadening of the vibrational wavepacket as plotted in Fig. 3i . It cannot be ruled out that this increased flexibility of the molecular bending mode contributes to a geometry change during the Auger lifetime. In the case of core-to-valence excitation of neutral acetylene [41] , Gadea et al. found that both the bending mode and isomerization to vinylidene stabilize the excited state. The singly charged core-excited ion created in a non-stationary state evolves during the core-hole lifetime. The momentum that the deuterium gains during the core-hole lifetime persists after the Auger decay. In addition, molecular geometry changes in the singly charged ion. This implies that Franck-Condon overlaps between the neutral and the dication will give a distorted estimate of the kinetic energy available for surmounting the isomerization barrier. In fact, it is necessary to account for both the geometry change and the acquired momentum during the core-hole lifetime when considering the Franck-Condon overlaps with the dicationic states. Hence, transition-state theory applied to the dication potential energy surface without accounting for the evolution during the core hole-lifetime is insufficient to describe the isomerization [2] , [3] , [4] , because the initial state excited by the core ionization is not static. The new class of time-resolved X-ray pump/X-ray probe experiments reported here enables direct probing of the molecular dynamics initiated by core ionization. By combining this technique with four-particle coincident detection, used for the first time at an X-ray FEL, we can monitor the evolving molecular geometry as a molecular movie. We applied this technique to a prototypical isomerization of the deuterated acetylene dication. We found that nonadiabatic interactions can couple nuclear motion into the electronic relaxation process in the first tens of femtoseconds following core ionization. In addition, it may be necessary to account for the geometry change that occurs during the core excitation to understand the early-time dynamics in core ionization of species that contain lighter nuclei. These findings have important implications for hydrocarbon isomerization and radiation damage by intense X-ray radiation. Experimental design This experiment was performed at the AMO beamline at LCLS in the High-Field Physics chamber, which is described in detail in ref. 10 . Pulses of X-ray radiation of 400 eV and up to 10 fs duration, 100 μJ per pulse, capable of core ionizing both the neutral- and doubly ionized C 2 D 2 , were used in both the pump and the probe steps. The average length of the electron bunches from which the X-ray pulses were generated was 10 fs, resulting in up to 10 fs long X-ray pulses. Simulations indicate that the duration of the photon pulse can be significantly shorter than the duration of the electron bunch [46] . Our experiment, which used non-resonant excitation, is insensitive to shot-to-shot fluctuations in X-ray pulse-frequency content. Two X-ray pulses with delays of 12, 25, 50 and 100 fs were derived from a single X-ray pulse using the split and delay apparatus described in ref. 47 . Briefly, the apparatus consists of two mirrors in which the pitch and height of one of the mirrors can be varied. The mirror splits the pulse into two pulses that intersect at a small-angle downstream. Adjusting one of the mirrors varies the difference in the path length between the two pulses and results in a variation of the time delay at the focus. In the nominal 0 fs time delay, only one X-ray pulse, but with twice the fluence as the pulses at other time delays, was delivered to the sample using one of the mirrors in the split and delay apparatus. The apparatus allows for sub-femtosecond precision in setting the delay. The two almost-collinear X-ray pulses intersect the molecular beam at a right angle. The approximate diameter of the focus was 50 μm 2 . The molecular beam was produced by expanding a 1:3 mixture of C 2 D 2 and He at a backing pressure of 2.4 bar through an Even-Lavie pulsed valve. The sample pressure, the distance of the nozzle from the interaction region and the photon intensity were adjusted such that, on average, only one molecule was fragmented per pump-probe event to realize unambiguous ion coincidence measurements. The data collection rate was 120 Hz. At each time delay, we analysed ∼ 2 × 10 6 events. After filtering out false coincidences, we analysed 1,087, 1,307, 1,137, 1,392 and 1,461 events at 0, 12, 25, 50 and 100 fs delay points, respectively. Ion fragments were extracted and accelerated towards the detector using a set of parallel plates in the direction perpendicular to both the molecular beam and X-ray pulses. The ions were detected using a microchannel plate combined with a three-layer delay-line anode detector (RoentDek Handles GmbH HexAnode). The voltages on the spectrometer plates were set to achieve the flat-field regime. The flat-field regime permitted a straightforward reconstruction of the particle momenta along the time-of-flight direction. The other two components of the momenta, in the plane of the detector, were reconstructed by implementing the advanced reconstruction technique [48] . This technique, described in ref. 48 , benefits from the redundancy of the ion impact information collected from the three detection layers. Momentum analysis To ensure that the fragments originated from the same parent ion, two constraints were applied in the impact analysis. The first constraint requires identification of all four C + /C + /D + /D + ions and up to two extra particles. The second constraint applies the conservation of momentum to the detected C + /C + /D + /D + coincidence so that the sum of the four momenta is close to zero in each direction in the lab frame individually. In other words: where D 1 , D 2 , C 1 , C 2 indicate the first and second deuterium and carbon atoms detected, and j is the lab frame-direction. The three lab frame directions, x , y , and z , refer to the direction of the molecular beam, the direction of the X-ray beam propagation and the time-of-flight direction. The value δp j is determined for each direction individually by identifying the width of the distribution of p j , which was 15 au, 28 au, and 92 au for the TOF and the two in-plane directions, respectively. The final ion fragment energy was scaled by a common factor of 0.9787 determined by a calibration with CO dissociative ionization. To make this calibration, we compared the measured energies of the 2 1 Σ + v =0 and v =1 peaks in the KER spectrum of core-ionized CO with those reported in the literature [49] . This scaling factor does not affect the momenta direction discussed in the manuscript. How to cite this article : Liekhus-Schmaltz, C. E. et al. Ultrafast Isomerization Initiated by X-Ray Core Ionization. Nat. Commun. 6:8199 doi: 10.1038/ncomms9199 (2015).